Interfacial assembly of dendritic microcapsules with host–guest chemistry The self-assembly of nanoscale materials to form hierarchically ordered structures promises new opportunities in drug delivery, as well as magnetic materials and devices. Herein, we report a simple means to promote the self-assembly of two polymers with functional groups at a water–chloroform interface using microfluidic technology. Two polymeric layers can be assembled and disassembled at the droplet interface using the efficiency of cucurbit[8]uril (CB[8]) host–guest supramolecular chemistry. The microcapsules produced are extremely monodisperse in size and can encapsulate target molecules in a robust, well-defined manner. In addition, we exploit a dendritic copolymer architecture to trap a small hydrophilic molecule in the microcapsule skin as cargo. This demonstrates not only the ability to encapsulate small molecules but also the ability to orthogonally store both hydrophilic and hydrophobic cargos within a single microcapsule. The interfacially assembled supramolecular microcapsules can benefit from the diversity of polymeric materials, allowing for fine control over the microcapsule properties. Molecular self-assembly is of importance in the fabrication of uniformly patterned functional surfaces, membranes and delivery vehicles, including hydrogels and microcapsules [1] , [2] . The self-assembly of molecular monolayers can be readily accomplished at a variety of interfaces, including metal (for example, gold), metal oxide substrates (for example, silica) or at an air–water interface, to form self-assembled monolayers [3] , [4] , [5] , [6] . More recently, the introduction of compartmentalization into such complex nano- or micro-scale systems is attracting considerable and wide-ranging interest for application in future delivery technologies [7] , [8] , [9] . Relative to planar interfaces, the spherical surface of a droplet offers improved interaction with the surrounding environment for sensing applications (for example, surface-enhanced Raman spectroscopy, SERS) or as a means of encapsulating a target cargo for localized study (for example, fluorescence resonance energy transfer, FRET) or protection (for example, enzymatic catalysis). The development of microfluidic techniques has revolutionised the formation of micro-scale droplets, allowing for high monodispersity in both size and composition, reproducibility, material efficiency and high throughput manipulation and analysis [10] , [11] . The self-assembly of nanoparticles at the droplet interface between immiscible fluids to form a Pickering emulsion, driven by a reduction in interfacial energy, is well-established [12] , [13] . Progressing to polymer-only materials to form multi-layer hollow structures promises new opportunities in drug delivery, as well as optical, acoustic, electronic and magnetic materials. However, polymer chain entanglement competes with thermal fluctuations and interfacial energy, giving rise to complicated self-assembly behaviour. To date, several approaches to prepare polymeric microcapsules have been adopted. In addition to self-assembled vesicles [14] , [15] , [16] , [17] , [18] or synthetic polymersomes [19] , the majority of reported structures rely on templating by exo [20] , [21] , [22] , meso [23] , [24] , endo [25] or exo–endo [26] , [27] methods. These approaches are experimentally laborious, with the use of a solid template requiring subsequent etching under relatively harsh conditions to obtain a hollow structure, lowering encapsulation and loading efficiencies. Droplets-in-droplet-based double or multiple emulsion strategies [28] , [29] , although powerful, depend on ingenious microfluidic devices and considerable interfacial tension between different phases. These assembles are typically not robust (for example, vesicles that cannot be dried) or more importantly rely on covalent crosslinking to give a microcapsule structure, limiting the opportunities for controlled disassembly required for on-demand release of cargo. While there have been examples of microcapsules formed from interfacial polymerization [30] , [31] or crosslinking [32] of monomers at the interface of a microdroplet, the interfacial assembly of pre-formed polymeric materials to form multi-layer amphiphilic microcapsules has not yet been demonstrated. Supramolecular host–guest chemistry has been applied in the preparation of various self-assembled structures, including polymers [33] , [34] , micelles [35] , hydrogels [36] , [37] , colloids [38] and more recently by our group, microcapsules [39] . In this supramolecular system, CB[8] was exploited to crosslink a naphthol (Np) modified poly(acrylamide) copolymer and methyl viologen (MV) functionalized gold nanoparticles, forming a nanocomposite supramolecular skin around aqueous microdroplets. CB[8] is a macrocyclic host molecule that is capable of simultaneously encapsulating two guests within its cavity, forming a stable yet dynamic ternary complex [40] , [41] . While we demonstrated a simple one-step approach to supramolecular microcapsules [39] , there were also a few limitations inherent to the system, such as the reliance on metal nanoparticles to direct self-assembly and the relatively large pore size, preventing encapsulation of small molecules. Initial attempts to replace the metal nanoparticles with polymeric equivalents resulted in all components dispersed throughout the aqueous phase, indicating that a new strategy towards the formation of supramolecular polymer-only microcapsules was required. Herein, we report the self-assembly of complementary-functionalized hydrophilic and hydrophobic copolymers that can be controllably brought together at the water–chloroform interface of a microfluidic droplet. By forming a robust ternary host–guest complex with CB[8], these functional copolymers can be reversibly crosslinked to form a polymeric skin at the microdroplet interface, giving rise to a supramolecular polymer-only microcapsule. These template free, interfacially assembled microcapsules are monodisperse in size and composition, with a high cargo encapsulation efficiency. Furthermore, we improve the efficacy of our microcapsule through the use of a dendritic copolymer. The dendritic nature of the functionalized copolymer enables the entrapment of small molecules within the microcapsule skin, demonstrating an additional level of compartmentalization of hydrophilic cargo (in this case) surrounding the microcapsule’s hydrophobic interior [42] , [43] . The extent of encapsulation by a dendritic copolymer, the ability to incorporate such a structure into the microcapsule skin and the subsequent triggered release of cargo via an external ultraviolet stimulus are presented. Interfacial assembly of supramolecular polymer capsules Supramolecular assembly between two complementary-functionalized polymers and CB[8] has been used to form a wide range of polymeric materials [35] , [44] , [45] . All of these examples to date, however, have taken place in aqueous media. By limiting each copolymer to distinct and immiscible phases, the assembly process can be restricted exclusively to the liquid–liquid interface, giving rise to a polymer sheet. Furthermore, by restricting the assembly to the spherical interface of a microdroplet a polymer microcapsule can be formed around the droplet, encapsulating its contents. Herein, we describe the preparation of microdroplets containing chloroform-in-water to template the interfacial assembly of the supramolecular microcapsules. A hydrophilic copolymer and CB[8] were dissolved in the aqueous continuous phase while a complementary hydrophobic copolymer was delivered in the chloroform microdroplet. Water-soluble poly(HEMA- co -StMV- co -FOA) ( P1 in Fig. 1b ) was synthesized by reversible addition-fragmentation chain-transfer (RAFT) polymerization containing 20 mol% of MV 2+ groups (weight average molecular weight (M w )=21 kDa, polydispersity (PDI)=1.3, Supplementary Fig. 1 ). Similarly, the hydrophobic poly(MMA- co -AA- co -HEMA) was synthesized via RAFT copolymerization (M w =16 kDa, PDI=1.2) and subsequently functionalized with naphthalene isocyanate and Rhodamine B isothiocyanate ( P2 in Fig. 1b and Supplementary Fig. 2 ). Interfacial assembly was accomplished using a microfluidic device comprising two inlets meeting at a single flow-focussing junction, as shown in Fig. 1a . To ensure generation of chloroform-in-water microdroplets, the surface of the microchannels were pretreated with a hydrophilic polyelectrolyte layer. At the microfluidic flow-focussing junction, the chloroform phase intersects with the perpendicularly flowing aqueous continuous phase, resulting in droplets of chloroform periodically being sheared ( Fig. 1c ). With a water/chloroform ratio of flow rates of 2:1, stable microdroplets were generated with a high level of monodispersity, as indicated by the narrow size distribution with a mean diameter of 102.4 μm and a low coefficient of variation of 1.6% ( Fig. 1d ). CB[8] can form a stable 1:1:1 heteroternary complex with an electron-deficient and electron-rich guest pair, such as a MV and a naphthol (Np) derivative, leading to an overall binding constant ( K a ) up to 10 12 M −2 in water [46] . Here the MV moiety is located on the hydrophilic copolymer P1 , while Np is found on the hydrophobic copolymer P2 . The aqueous solution contained 60 μM of the MV dication (MV 2+ ) pendant group and 60 μM CB[8], while the dispersed phase consisted of a chloroform solution containing 60 μM of naphthalene moieties. 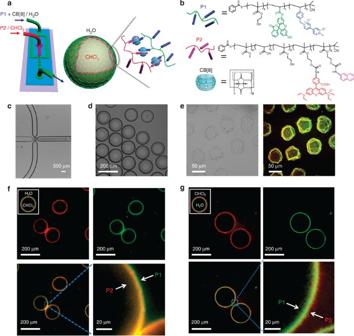Figure 1: Supramolecular assembly of microcapsules at the interface of microfluidic droplets. (a) Schematic representation of the microdroplet generation process using a microfluidic flow-focussing device, where an aqueous continuous phase containing CB[8] and copolymerP1(functionalized with MV and FOA) intersects an immiscible chloroform phase containing copolymerP2(functionalized with Np and Rhodamine B), at a flow-focussing microchannel junction to form a periodic flow of oil-in-water microdroplets. (b) The chemical structures of hydrophilic poly(HEMA-co-StMV-co-FOA),P1; hydrophobic poly(MMA-co-AA-co-HEMA-NP),P2and CB[8]. (c) Micrograph of oil-in-water microdroplets generated at the microfluidic flow-focussing channel junction. (d) The high monodispersity of the formed microdroplets is demonstrated by the narrow size distribution (d=102.4±0.5 μm). (e) Bright field (left) and fluorescence (right) images of microcapsules formed after evaporation of the chloroform droplet, resulting in a collapsed capsule-like structure. (f) Fluorescence micrographs of the highly monodisperse chloroform-in-water microdroplets, demonstrating the interfacial assembly ofP2(rhodamine tagged, red) within the droplet andP1(fluorescein tagged, green) present in the external media. (g) Fluorescence micrographs of the inverted water-in-chloroform microdroplets, illustrating reversal ofP1andP2at the droplet interface. Figure 1: Supramolecular assembly of microcapsules at the interface of microfluidic droplets. ( a ) Schematic representation of the microdroplet generation process using a microfluidic flow-focussing device, where an aqueous continuous phase containing CB[8] and copolymer P1 (functionalized with MV and FOA) intersects an immiscible chloroform phase containing copolymer P2 (functionalized with Np and Rhodamine B), at a flow-focussing microchannel junction to form a periodic flow of oil-in-water microdroplets. ( b ) The chemical structures of hydrophilic poly(HEMA- co -StMV- co -FOA), P1 ; hydrophobic poly(MMA- co -AA- co -HEMA-NP), P2 and CB[8]. ( c ) Micrograph of oil-in-water microdroplets generated at the microfluidic flow-focussing channel junction. ( d ) The high monodispersity of the formed microdroplets is demonstrated by the narrow size distribution ( d =102.4±0.5 μm). ( e ) Bright field (left) and fluorescence (right) images of microcapsules formed after evaporation of the chloroform droplet, resulting in a collapsed capsule-like structure. ( f ) Fluorescence micrographs of the highly monodisperse chloroform-in-water microdroplets, demonstrating the interfacial assembly of P2 (rhodamine tagged, red) within the droplet and P1 (fluorescein tagged, green) present in the external media. ( g ) Fluorescence micrographs of the inverted water-in-chloroform microdroplets, illustrating reversal of P1 and P2 at the droplet interface. Full size image The heteroternary complex exclusively forms at the interface of the microdroplet between P1 ·CB[8] and P2 , leading to the interfacial formation of a supramolecular polymeric skin ( P2 in · P1 out ⊂ CB[8]). The inner chloroform phase of the microdroplet can be evaporated, allowing the microcapsule skin to be visualized. As the droplet evaporates, the diameter contracted, up to 120 s, at which point the spherical shape of the droplet became slightly distorted. As evaporation proceeded, wrinkles in the surface became visible, with these developing into marked creases and eventually folds. The appearance of wrinkling is used as evidence that an elastic polymer skin has formed at the interface of the droplet and we are no longer in a liquid–liquid regime. Upon further evaporation, the droplet can no longer support the microcapsule skin, resulting in the top of the microcapsule collapsing onto the base, giving rise to sharp, irregular folds once dry ( Fig. 1e ). The observed collapse of the microcapsule, rather than ingress of the carrier fluid to replace the lost droplet media, is attributed to surfactant coating the capsule skin and acting as a barrier. Fluorescent microscopy of the microcapsule shell showed a bilayer of polymers that comprised the supramolecular self-assembled network. Green fluorescence from flurorescein-labelled P1 can be clearly resolved on the outer layer of the polymeric shell, while the chloroform droplet-bound P2 (Rhodamine B labelled, red) is completely localized at the inside face of the microcapsule ( Fig. 1f ). The absence of any fluorescence dispersed across either the droplet or carrier solvent (water) confirms the quantitative nature of this interfacial templating effect, with all functionalized copolymers localized within the resultant microcapsule skin. To assess the significance of the supramolecular heteroternary complex, a number of control experiments were carried out. In the absence of CB[8], as shown in Fig. 2a , formation of stable microcapsules was not observed, rather any structures formed were observed to break, giving rise to flower-like polymer sheets. Similarly, microcapsule formation was not observed when employing the smaller macrocycle cucurbit[7]uril (CB[7]), which is capable of complexing only one MV 2+ moiety, but not a second guest, preventing formation of a 1:1:1 heteroternary complex. In this case, copolymers P1 and P2 were no longer assembled at the chloroform–water droplet interface, but instead remained dispersed throughout the media as shown in Fig. 2b . Importantly, both of these control experiments show that the aggregation of supramolecular copolymers exclusively occurs at the droplet interface as a direct result of CB[8] heteroternary complex formation. 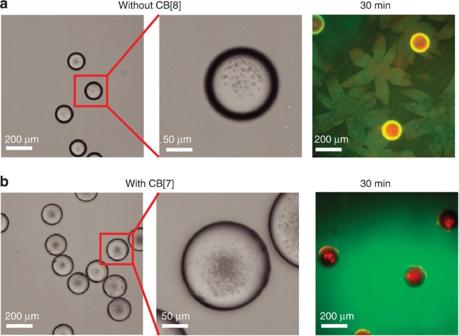Figure 2: Confirmation of the role of supramolecular crosslinking in microcapsule formation. (a) Microdroplets formed in the absence of CB[8] did not lead to the formation of robust microcapsules, any microcapsules that did form were observed to rupture, giving rise to flower-like polymer sheets. (b) Similarly, attempts to form microcapsules via CB[7] were unsuccessful, with fluorescence microscopy confirming that copolymersP1andP2were no longer assembling at the chloroform–water droplet interface, but instead remained dispersed throughout the media. Figure 2: Confirmation of the role of supramolecular crosslinking in microcapsule formation. ( a ) Microdroplets formed in the absence of CB[8] did not lead to the formation of robust microcapsules, any microcapsules that did form were observed to rupture, giving rise to flower-like polymer sheets. ( b ) Similarly, attempts to form microcapsules via CB[7] were unsuccessful, with fluorescence microscopy confirming that copolymers P1 and P2 were no longer assembling at the chloroform–water droplet interface, but instead remained dispersed throughout the media. Full size image To further demonstrate the versatility of this interfacial approach to supramolecular microcapsule formation, the inverse ‘water-in-chloroform’ microdroplets were prepared in the corresponding hydrophobic microfluidic flow-focussing device. The nature of the continuous and discontinuous phases were reversed, with P1 and CB[8] now confined to the aqueous droplet and P2 located in the organic carrier fluid (1:5 v/v mixture of hexadecane in chloroform). As before, all polymeric materials localized at the microdroplet interface for supramolecular assembly, with the complementary fluorescence profile observed as highlighted in Fig. 1g , with P1 now visible on the inner face and P2 on the outside ( P1 in · P2 out ⊂ CB[8]). Interfacial assembly of dendritic supramolecular capsules To demonstrate how this multi-layer microcapsule can be exploited for both cargo encapsulation and subsequent release with an external stimuli, such as ultraviolet light, a dendritic copolymer was designed and synthesized via RAFT copolymerization of divinyl monomer, ethylene glycol dimethacrylate (EGDMA), containing a ultraviolet-responsive azobenzene-containing second guest for CB[8] ( Fig. 3 ). 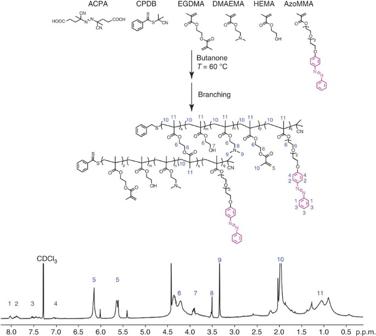Figure 3: Chemical structures and1H NMR spectrum of dendritic copolymer H1. The dendritic copolymer (H1) was synthesized via RAFT copolymerization of the divinyl monomer, ethylene glycol dimethacrylate (EGDMA), and incorporates azobenzene for photoresponsive complexation with CB[8]. The branching ratio is defined as the ratio of EGDMA units to all monomer units, as shown inSupplementary Equation 1. Figure 3: Chemical structures and 1 H NMR spectrum of dendritic copolymer H1. The dendritic copolymer ( H1 ) was synthesized via RAFT copolymerization of the divinyl monomer, ethylene glycol dimethacrylate (EGDMA), and incorporates azobenzene for photoresponsive complexation with CB[8]. The branching ratio is defined as the ratio of EGDMA units to all monomer units, as shown in Supplementary Equation 1 . Full size image Two vinyl groups exist within the EGDMA monomer that can form a branch point under the right synthetic conditions, thus yielding a dendritic architecture (instead of a crosslinked network) using controlled/living free radical polymerization [47] , [48] . During copolymerization towards the dendritic polymer, poly(EGDMA- co -DMAEMA- co -HEMA- co -Azo), ( H1 ) was monitored by tetrahydrofuran gel permeation chromatography (THF-GPC) (refractive index detector, Supplementary Fig. 3 ), which indicated a broadening of peaks between 1 h (PDI=2.3) and 3 h (PDI=4.2). Complete solubility (in THF) with concommitant peak broadening suggested that the major reaction pathway up to 3 h was the combination of growing polymer chains achieving a dendritic structure. The molecular weight of the purified polymer H1 reached 41.8 kDa (PDI=2.7) at 3 h without gelation ( Supplementary Table 1 ). H1 displayed a high branching ratio of 17.5% and contained 2.5 mol% of azobenzene guest, as calculated from the 1 H nuclear magnetic resonance (NMR) spectrum ( Fig. 3 ), indicating a highly branched structure formed from enhanced intermolecular coupling rather than chain growth. Here the branching ratio is defined as the proportion of branched EGDMA monomers relative to the sum of all monomer units, including linear EGDMA, branched EGDMA, HEMA, DMAEMA and AzoMMA monomers (see Supplementary Equation 1 for calculation). Dendritic copolymer H1 was able to entrap hydrophilic small molecule ‘cargo’ on account of its unique three-dimensional nanoscale structure. Here the fluorescent dye, Congo Red (CR), was encapsulated ( Fig. 4a ) for subsequent studies. The dendritic copolymer is far superior in its ability to entrap small molecules over its linear analogue as demonstrated by a control experiment using poly(MMA- co -DMAEMA- co -HEMA- co -Azo), with a comparable molecular weight, M w =38.1 kDa and PDI=1.4. The absorption studies concluded that the dendritic H1 can entrap 4.1 times more CR into a hydrophobic environment than its linear analogue, at the same concentration of copolymer ( Fig. 4a , Supplementary Table 2 and Supplementary Fig. 5 ). To fabricate dendritic supramolecular microcapsules via interfacial assembly, monodisperse chloroform microdroplets containing CR entrapped within H1 were generated in an aqueous continuous phase, which contained P1 and CB[8] ( Fig. 4b ). It is worth noting that although H1 does not contain a fluorescent tag, the entrapped fluorescent dye, CR, was used to directly monitor polymer assembly at the droplet interface. It was observed by fluorescent microscopy that interfacial assembly indeed occurred at the droplet interface ( Fig. 4c ), leading to supramolecular microcapsule formation upon subsequent evaporation of the chloroform, with the formation of creases and folds upon collapse of the flexible polymer skin ( Fig. 4d,e ). Microdroplets generated in the absence of CB[8] did not lead to robust aggregation at the droplet interface, leading to the formation of dense polymer beads of H1 upon evaporation ( Fig. 4f ). 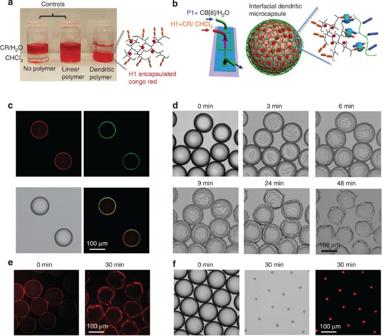Figure 4: Interfacial assembly of supramolecular dendritic microcapsules. (a) Photograph of the entrapment of water-soluble CR and its transfer into organic solvent by the dendritic copolymer,H1. (b) Schematic representation of the microdroplet generation process using a microfluidic flow-focussing device, comprising an aqueous continuous phase containing CB[8] andP1, intersecting a perpendicular flow of chloroform containing dendritic copolymerH1with entrapped CR to form chloroform-in-water microdroplets. (c) Fluorescence and optical micrographs of the highly monodisperse microdroplets formed, illustrating the interfacial assembly of an innerH1layer (entrapped CR) and aP1outer layer (fluorescein tagged). (d) Bright field images of the formation of the microcapsule skin as the chloroform microdroplet evaporates, resulting in a collapsed capsule-like structure. (e) Fluorescence images of microcapsule formation verifying that CR is entrapped within the microcapsule wall. (f) A control experiment in the absence of CB[8], confirmed thatP1andH1no longer assemble at the interface of the droplets, but remain dispersed within the media to form dense polymer beads ofH1upon evaporation, rather than a microcapsule. Figure 4: Interfacial assembly of supramolecular dendritic microcapsules. ( a ) Photograph of the entrapment of water-soluble CR and its transfer into organic solvent by the dendritic copolymer, H1 . ( b ) Schematic representation of the microdroplet generation process using a microfluidic flow-focussing device, comprising an aqueous continuous phase containing CB[8] and P1 , intersecting a perpendicular flow of chloroform containing dendritic copolymer H1 with entrapped CR to form chloroform-in-water microdroplets. ( c ) Fluorescence and optical micrographs of the highly monodisperse microdroplets formed, illustrating the interfacial assembly of an inner H1 layer (entrapped CR) and a P1 outer layer (fluorescein tagged). ( d ) Bright field images of the formation of the microcapsule skin as the chloroform microdroplet evaporates, resulting in a collapsed capsule-like structure. ( e ) Fluorescence images of microcapsule formation verifying that CR is entrapped within the microcapsule wall. ( f ) A control experiment in the absence of CB[8], confirmed that P1 and H1 no longer assemble at the interface of the droplets, but remain dispersed within the media to form dense polymer beads of H1 upon evaporation, rather than a microcapsule. Full size image The CB[8] heteroternary complex, beyond providing a means for directing self-assembly and locking together the multi-layer capsule skin, also imparts inherent stimuli responsiveness that can be employed to trigger the release of encapsulants. This is demonstrated here through photoisomerization of the azobenzene moiety on H1 , destabilizing the heteroternary complex and leading to capsule disassembly. As synthesized, the azobenzene group on H1 exists primarily as the trans -isomer, however, upon irradiation with ultraviolet light (365 nm) it photoisomerizes into the cis -isomer ( Fig. 5a left) [49] , with the photo-stationary state expected to contain up to 80% of the cis -isomer in the presence of CB[8] ref. 33 . This conformational change ( Fig. 5a right) does not allow for heteroternary complexation within the cavity of CB[8]. This leads to significant disassembly of the microcapsule skin, resulting in a rapid increase in porosity and liberation of individual dendritic polymer, allowing the CR to partition into the aqueous phase over time ( Fig. 5b ). Consequently, ultraviolet stimulus-controlled release of the CR cargo from P1 out · H1 in × CR ⊂ CB[8] microcapsules was achieved after brief exposure to ultraviolet light (120 s), which could be observed in the surrounding aqueous media over time. To avoid any evaporation of the chloroform from the microcapsules, they were collected in a covered vial while the release behaviour of CR was measured. Our experimental results showed that exposure to ultraviolet light for 120 s led to facile disruption of the capsule, giving rise to a steady release of the fluorescent cargo, with 33% released in 40 min. In contrast, a negligible release of cargo was observed for the control experiment over a similar timescale, with the remaining CR localized within the microcapsule skin ( Fig. 5c ). 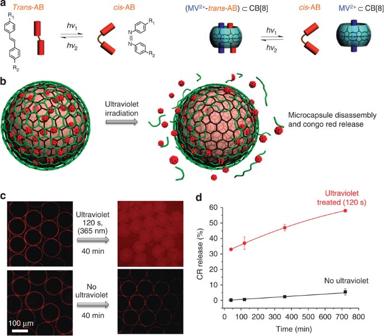Figure 5: Photo-triggered release of cargo from supramolecular dendritic microcapsules. (a) Ultraviolet light-driven photo-isomerization of the azobenzene moiety can be used to disassemble the heteroternary supramolecular complex between MV, azobenzene and CB[8]. (b) Schematic representation of the triggered disassembly of theH1-containing microcapsule on exposure to 365 nm ultraviolet light with corresponding release of the entrapped CR molecular cargo. (c) Fluorescence micrographs showing release of the entrapped CR fromH1·P1⊂CB[8] microcapsules, with and without initial ultraviolet irradiation. (d) Time-resolved CR release profiles fromH1·P1⊂CB[8] microcapsules as a function of initial ultraviolet irradiation for 120 s. Figure 5d depicts the long-term release profile of CR from the dendritic supramolecular microcapsules with and without initial ultraviolet irradiation for 120 s. Over 12 h, microcapsules that had been irradiated slowly released up to 60% of their cargo, compared with only 5% for the unexposed control. Figure 5: Photo-triggered release of cargo from supramolecular dendritic microcapsules. ( a ) Ultraviolet light-driven photo-isomerization of the azobenzene moiety can be used to disassemble the heteroternary supramolecular complex between MV, azobenzene and CB[8]. ( b ) Schematic representation of the triggered disassembly of the H1 -containing microcapsule on exposure to 365 nm ultraviolet light with corresponding release of the entrapped CR molecular cargo. ( c ) Fluorescence micrographs showing release of the entrapped CR from H1 · P1 ⊂ CB[8] microcapsules, with and without initial ultraviolet irradiation. ( d ) Time-resolved CR release profiles from H1 · P1 ⊂ CB[8] microcapsules as a function of initial ultraviolet irradiation for 120 s. Full size image We have shown a simple and robust means of directing the assembly of supramolecular polymeric materials at a hydrophilic/hydrophobic droplet interface to form an encapsulating skin. The interfacial assembly process critically relies upon the supramolecular heteroternary host–guest complex formed between CB[8] and suitable guest moieties on the constituent copolymers. This bilayer assembly of hydrophilic and hydrophobic copolymers will uniquely allow for the expression of orthogonal chemical functionalities at the inner and outer faces of the microcapsule, enabling greater control over the properties of the microcapsule. By moving from a nanoparticle-mediated microcapsule assembly process to one driven by interfacial assembly of copolymers, we retain the advantages of supramolecular assembly, but benefit from the diversity of synthesized polymeric materials, allowing for fine control over the properties and function of the microcapsules, including wall thickness, permeability and an expanded toolset for cargo release. By exploiting a dendritic copolymer, small molecules were successfully encapsulated, overcoming the restriction of molecular weight. Combined with the ability to segregate and store water-soluble and oil-soluble cargo within a single structure, this extends the range of potential application into new areas, such as drug delivery. The incorporation of azobenzene as a polymer-bound guest for CB[8] enabled the introduction of a controllable release valve into the microcapsule skin, demonstrating remote manipulation of microcapsule properties under mild conditions. Importantly, these interfacially assembled bilayer microcapsules afford a unique platform with which one could quantitatively investigate the mechanism and kinetics of self-assembly at liquid–liquid or soft matter interfaces, which is of great relevance in all biological systems [50] , [51] . Materials Methyl methacrylate (MMA), hydroxyethylmethacrylate, EGDMA, N,N-dimethylaminoethyl methacrylate and acrylic acid (AA) monomers were purchased from Sigma-Aldrich and were passed through a column of silica gel and purged with high purity nitrogen for 1 h prior to use. Fluorescein o -acrylate (FOA) and 2-naphthyl isocyanate were purchased from Alfa Aesar. 2-Cyano-2-propyl benzodithioate, 4,4'-azobis(4-cyanovaleric acid) (ACPA), Rhodamine B isothiocyanate, CR (analytical standard), polyvinyl acetate (M w =13–23 kDa) and 2-butanone (HPLC grade) were purchased from Sigma-Aldrich. MV-styrene, the azobenzene monomer and CB[8] were synthesized as previously reported (See Supplementary Methods ). Solvents and reagents were used without further purification unless otherwise stated. Preparation of poly(HEMA- co -StMV- co -FOA) (P1) Poly(HEMA- co -StMV- co -FOA) was synthesized via RAFT polymerization using the unmodified chain transfer agent 2-cyano-2-propyl benzodithioate. To a two-neck round bottom flask were added 2-cyano-2-propyl benzodithioate (CPBD, 22.1 mg, 0.1 mmol, 1 equiv. ), hydroxyethylmethacrylate (HEMA, 1.3 g, 10 mmol, 100 equiv. ), MV-styrene (StMV, 0.9 g, 2 mmol, 20 equiv.) and FOA (38.6 mg, 0.1 mmol, 1 equiv.) in a 50:50 wt% mixture of aqueous methanol (6 ml). Oxygen was removed by bubbling argon through the solution for 20 min, followed by the subsequent addition of ACPA (14 mg, 0.05 mmol, 0.5 equiv.). The flask was then immersed in a preheated oil bath (65 °C) and the solution was stirred at 400 r.p.m. for 24 h. The resultant polymer was dialysed in water through a MWCO 6,000–8,000 membrane and freeze dried. The formed polymer was characterized to give M w =21 kDa, PDI=1.2 from GPC, and HEMA/StMV=100:23 from 1 H NMR ( Supplementary Fig. 1 ). Preparation of poly(MMA- co -AA- co -HEMA-Np) (P2) Poly(MMA- co -AA- co -HEMA-Np) was synthesized via RAFT polymerization using the unmodified chain transfer agent CPBD. To a two-necked round bottom flask were added CPBD (22.1 mg, 0.1 mmol, 1 equiv. ), MMA, 1.0 g, 10 mmol, 100 equiv. ), HEMA (0.325 g, 2.5 mmol, 25 equiv.) and AA (0.18 g, 2.5 mmol, 25 equiv.) in 2-butanone (8 ml). Oxygen was removed by bubbling argon through the solutions for 20 min, followed by the subsequent addition of ACPA (14 mg, 0.05 mmol, 0.5 equiv.). The flask was immersed in a preheated oil bath (65 °C) and the solution stirred at 400 r.p.m. for 24 h. The polymer was precipitated into cold hexane and finally dried in vacuo at 50 °C. The resultant polymer was then subsequently functionalized with naphthalene isocyanate (10% molar ratio) and Rhodamine B isothiocyanate (1% molar ratio). The final polymer was characterized to give M w =16 kDa, PDI=1.2 from GPC, MMA/HEMA/AA/Np=100:30:27.2:4.5 from 1 H NMR ( Supplementary Fig. 2 ). Preparation of dendritic poly(EGDMA- co -DMAEMA- co -HEMA- co -Azo) (H1) Poly(EGDMA- co -DMAEMA- co -HEMA- co -Azo) was synthesized via RAFT polymerization using the unmodified chain transfer agent CPBD. To a two-neck round bottom flask were added CPBD (22.1 mg, 0.1 mmol, 1 equiv. ), EGDMA (3.98 g, 20 mmol, 200 equiv. ), HEMA (0.35 g, 2.5 mmol, 25 equiv. ), DMAEMA (0.39 g, 2.5 mmol, 25 equiv.) and AzoMMA (199 mg, 0.5 mmol, 5 equiv.) in 2-butanone (12 ml, [EGDMA]=1.25 M). Oxygen was removed by bubbling argon through the solutions for 20 min, followed by the subsequent addition of ACPA (14 mg, 0.05 mmol, 0.5 equiv.). The flask was immersed in a preheated oil bath (60 °C) and the solution stirred at 400 r.p.m. for the desired reaction time. The resultant polymer was precipitated into cold hexane and dried in vacuo at room temperature. The purified polymer was characterized to give M w =41.8 kDa, PDI=2.7 from GPC ( Supplementary Table 1 and Supplementary Fig. 3 ), linear EGDMA/branched EGDMA/HEMA/DMAEMA/AzoMMA=35:17.5:21:24:2.5 from 1 H NMR ( Fig. 3 and Supplementary Equation 1 ). Encapsulation of CR Typically, 2 ml of an aqueous solution of CR (0.01 mg ml −1 ) was mixed with 2 ml of a chloroform solution containing the dendritic polymer H1 in a glass vial and the mixture was shaken for 24 h to ensure the two phases were sufficiently mixed. The two phases were allowed to separate and the lower chloroform layer was transferred to a cuvette and its absorption spectrum was recorded. In all experiments, the concentration of CR in the aqueous phase was in great excess to ensure the maximum loading capacity (C load ) within H1 was achieved. The amount of encapsulated dye was determined quantitatively from the absorption spectrum (CR λ max =498 nm). Detailed results are presented in Supplementary Table 2 for the ability of the dendritic polymer H1 to encapsulate CR compared with the equivalent linear polymer, poly(MMA- co -DMAEMA- co -HEMA- co -Azo), as a control (see Supplementary Information ). The calibration of absorbance against CR concentration is shown in Supplementary Fig. 4 . Fabrication and characterization of the microcapsules All microfluidic chips used in this work were manufactured from silica and purchased fully assembled from Dolomite. To produce monodisperse oil-in-water microdroplets, a hydrophilic flow-focussing microfluidic chip was employed (100 μm channel depth, 3000158 Droplet Junction Chip), and to ensure a hydrophilic microchannel the chip was pretreated with a sequential layer-by-layer deposition of polyallylamine hydrochloride and poly(sodium styrene sulfonate) polyelectrolytes. The hydrophobic phase (chloroform) and the hydrophilic aqueous phase were injected into the microfluidic device via two syringe pumps (PHD, Harvard Apparatus) with controlled flow rates. The continuous aqueous phase was prepared by dissolving CB[8] and P1 in a 1 wt% polyvinylalcohol solution, while the discontinuous phase comprised of a 4:1 v/v mix of chloroform and HFE-7500 (3M), into which P2 was dissolved. Microdroplet formation was initiated by first pumping the aqueous continuous phase into the device at the rate of 400 μl h −1 , to fill the appropriate channels, followed by the discontinuous oil phase into the middle channel of the flow-focussing device at 200 μl h −1 . At these flow rates, the oil flow was periodically sheared at the flow focus to form microdroplets within an aqueous carrier flow. For a typical experiment, the concentrations of MV, Np and CB[8] were all 30 μM. Once formed microdroplets were collected on the surface of glass slide for further study. To prepare the inverse water-in-oil microdroplet, the equivalent hydrophobic flow-focussing microfluidic chip was employed (190 μm etch depth, 3000437 Droplet Junction Chip). As before, the two phases were injected into the microfluidic device via syringe pumps with precise control over the flow rate. The discontinuous phase was prepared by dissolving copolymer P1 and CB[8] in water, while the continuous oil phase comprised a 1:5 v/v mixture of chloroform in hexadecane, into which P2 was dissolved. To prevent fusion of the prepared microdroplets, 2 wt% of the surfactant Span 80 was further added to the continuous phase. As before, the continuous phase (oil) was first pumped into the device at the rate of 400 μl h −1 to fill the appropriate channels followed by the aqueous discontinuous phase at 200 μl h −1 . At these flow rates, the aqueous flow was periodically sheared at the flow focus to form water-in-oil microdroplets. In a typical experiment, the concentrations of MV, Np and CB[8] were all 30 μM. Once formed, microdroplets were collected on the surface of glass slide for further study. CR loaded microdroplets, formed from dendritic polymer H1 , were templated via an oil-in-water microdroplet motif and as such required a hydrophilic microfluidic channel. As before, the continuous aqueous phase was prepared by dissolving CB[8] and P1 in 1 wt% polyvinylalcohol solution, however the discontinuous phase contained H1 carrying CR dissolved in chloroform exclusively. Microdroplet formation was initiated by first pumping the aqueous continuous phase into the device at the rate of 400 μl h −1 , to fill the appropriate channels, followed by the discontinuous oil phase into the middle channel of the flow-focussing device at 200 μl h −1 . At these flow rates, the oil flow was periodically sheared at the flow focus to form microdroplets within an aqueous carrier flow. In a typical experiment, the concentrations of MV, Azo and CB[8] were all 150 μM. Once formed, microdroplets were collected on the surface of glass slide for further study. Ultraviolet-triggered microcapsule disassembly and cargo release To investigate triggered disassembly of the supramolecular crosslinks, leading to microcapsule rupture, the fluorescent dye, CR, was employed to probe release of encapsulant from the microcapsule. Throughout the release experiment, the vial was kept in the dark and at room temperature to minimize reconversion back to the trans -isomer. In addition, the presence of polyvinyl acetate in the carrier solution stabilized the chloroform droplets throughout the release studies. The dendritic polymer ( H1 ) was used to entrap CR as described above, with 3.64 mg polymer H1 found to contain 1.82 μg of CR (0.05 wt% loading) and then employed in the preparation of microcapsules, with CR encapsulated within the microcapsule skin. After washing the formed microcapsules three times with water to remove any free dye, 2.5 ml of water was added into the vial. The prepared microcapsules were exposed to a ultraviolet light source using a LZC-ORG photo-reactor with both 350 nm wavelength lamps for 2 min. Aliquots of the aqueous phase were collected at set intervals after the initial ultraviolet exposure (40, 120, 360 and 720 min) and the absorption spectrum recorded. The release profile of CR from the microcapsules after ultraviolet exposure and for a control are given in Supplementary Table 3 and Fig. 5 . Instrumentation 1 H NMR spectra (400 MHz) were collected on a Bruker Avance QNP 400 MHz Ultrashield spectrometer, equipped with a 5-mm BBO ATM probe with a z-gradient. Ultraviolet/visible spectra were recorded on a Varian Cary 4000 UV/visible spectrophotometer. Microscopic images and fluorescence images were obtained using an Olympus IX81 inverted optical microscope coupled with a camera of Andor Technology EMCCD iXonEM+ DU 897. Photoirradiation was performed on a LZC-ORG photoreactor with both 365 nm wavelength lamps. Titration experiments were carried out on a ITC200 from Microcal Inc. M w , number average molecular weight (M n ) and polydispersity (M w /M n ) were obtained by aqueous or THF-GPC. The aqueous GPC setup consisted of a Shodex OHpak SB column, connected in series with a Shimadzu SPD-M20A prominence diode array detector, a Wyatt DAWN HELEOS multi-angle light scattering detector and a Wyatt Optilab rEX refractive index detector. The THF GPC setup consisted of two 30-cm PLgel Mixed-C columns in series, eluted using THF and calibrated against a series of 12 near-monodisperse PMMA standards (M p from 690 to 1,944,000 g mol −1 ). The polymers were analyzed in THF at a concentration of 5.0 mg ml −1 . All calibrations and analysis were performed at 35 °C at a flow rate of 1 ml min −1 . How to cite this article : Zheng, Y. et al . Interfacial assembly of dendritic microcapsules with host–guest chemistry. Nat. Commun. 5:5772 doi: 10.1038/ncomms6772 (2014).